Rapid one-step18F-radiolabeling of biomolecules in aqueous media by organophosphine fluoride acceptors Currently, only a few 18 F-radiolabeling methods were conducted in aqueous media, with non-macroelement fluoride acceptors and stringent conditions required. Herein, we describe a one-step non-solvent-biased, room-temperature-driven 18 F-radiolabeling methodology based on organophosphine fluoride acceptors. The high water tolerance for this isotope-exchange-based 18 F-labeling method is attributed to the kinetic and thermodynamic preference of F/F over the OH/F substitution based on computational calculations and experimental validation. Compact [ 18/19 F]di- tert -butyl-organofluorophosphine and its derivatives used as 18 F-labeling synthons exhibit excellent stability in vivo. The synthons are further conjugated to several biomolecular ligands such as c(RGDyk) and human serum albumin. The one-step labeled biomolecular tracers demonstrate intrinsic target imaging ability and negligible defluorination in vivo. The current method thus offers a facile and efficient 18 F-radiolabeling pathway, enabling further widespread application of 18 F. Positron emission tomography (PET) is a highly sensitive, quantitative, noninvasive imaging technique, and therefore is one of the most popular imaging modalities for disease diagnosis and monitoring of therapeutic effects [1] . The 18 F-radionuclide contributes greatly to the success of this imaging method and is often preferred for PET imaging due to its wide availability, favorable half-life (109.8 min), high isotopic purity, and low positron energy (640 keV), allowing sequential acquisition of PET images with a relatively high resolution [2] . However, to synthesize 18 F-labeled PET tracers, traditional labeling methods are mostly based on carbon-fluorine bond formation, which usually demands multiple steps and/or harsh reaction conditions such as heating at high temperatures in organic media [3] . Moreover, most 18 F-radiolabeling reactions require strict anhydrous conditions due to the limited reactivity of the fluoride anion as a nucleophile in aqueous solution [4] (Fig. 1a ). Feasible and efficient 18 F-labeling methods in physiological media remain highly desirable for the introduction of 18 F into useful biomolecules, such as water-soluble peptides and antibodies that bind to overexpressed receptors in various inflammatory tissues and tumors [2] . Fig. 1 Overview of 18 F-labeling methods for solvent/heat-sensitive biomolecules. a Commonly used multistep synthetic route beginning with drying of aqueous [ 18 F]F − . b One-step 18 F-labeling of biomolecules via an organophosphine fluoride acceptor that allows for efficient labeling with good RCYs (>50%) under mild conditions within 5–15 min Full size image A few studies [5] , [6] , [7] , [8] reported that fluorinase enzyme can catalyze the incorporation of 18 F into PET radiotracers under aqueous conditions. However, the high substrate specificity severely limits the scope of application for this enzyme method [7] . Several direct aqueous 18 F-labeling approaches have been reported, using organofluorosilicons [2] , [9] , [10] , [11] , [12] , [13] , [14] , [15] , aluminum complexes [16] , [17] , [18] , [19] or trifluoroborates [20] , [21] , [22] , [23] , [24] , [25] , [26] , [27] , [28] as non-carbon fluoride acceptors to afford one-step labeling of peptides. These non-macroelement fluoride acceptor-based methods exploit their Lewis acid characteristics. Lewis acid promoters, such as SnCl 4 and AlCl 3 , are sometimes required to activate the fluorine-element bond to facilitate [ 18 F]F¯ incorporation in these systems [29] . The high bond enthalpy and low activation energy for the binding of Si, Al, and B with F − lead to the formation of stable bonds with 18/19 F − instead of being attacked by and bonded with OH − [30] . However, these methods still pose obvious drawbacks: (i) limited stability and high lipophilicity of the organosilicon-based 18 F-labeling blocks; (ii) specific pH requirement for trifluoroborate-based 18 F-labeling; (iii) steric effect of bulky Al- 18 F-based chelate synthons; and iv) potential biosafety issue due to possible metal contamination in the final product. Recently, a bulky [GaF 3 (BnMe 2 -tacn)], another metal chelate system, was labeled in aqueous solutions by 18 F/ 19 F isotopic exchange but showing slight defluorination of the 18 F-labeled product in plasma [29] . Collectively, non-solvent-biased 18 F-labeling methods with macroelement-composed fluoride acceptors remain unexplored. The phosphorus (P) element is essential for life and phosphines are components of deoxyribonucleic acid, ribonucleic acid, adenosine triphosphate, and phospholipids [31] . The formation heat of phosphine fluoride radicals is −12.5 ± 5 kcal mol −1 while those of silicon fluoride, boron fluoride, and fluorocarbon radicals are −4.8 ± 3, −27.7 ± 3.3, and 61.0 ± 2 kcal mol −1 , respectively [32] . Therefore, phosphorus, boron, and silicon readily form more stable products with fluorine (compared to fluorocarbon). Phosphorus is strongly fluorophilic based on previous reports [33] , [34] . For example, the affinity of F-P in PF 5 (380 kJ mol −1 ) is even higher than that in F-B in BF 3 (346 kJ mol −1 ). Preparation of compounds containing the P- 18 F bond was demonstrated by 18 F-labeling of phospho-pesticide [35] and NCH-PF 5 [33] in organic solvents under heating condition. Here we rationally design and develop organophosphine precursors that allow for easy synthesis and efficient radiolabeling with high radiochemical yields (RCYs) and molar activities under mild conditions. In this way, 18 F-labeled biomolecules are successfully obtained in either organic solvents or aqueous media with high RCY up to 100% within 15 min, as shown in Fig. 1b . Proof-of-concept of 18 F-labeling with heat/solvent-sensitive biomolecules in one step is demonstrated by biomolecular tracers include 18 F-labeled human serum albumin (HSA) for blood pool imaging and 18 F-labeled c(RGDyk) which targets the integrin α v β 3 receptor of the U87MG cell (glioblastoma). Thus, the method reported here permits non-specialist-manageable rapid 18 F-labeling of extensive biomolecules and their use in PET imaging. Mechanism of rapid H 2 O-resistant 18 F/ 19 F exchange We first performed computational density functional theory (DFT) calculations to simulate the F/F isotope exchange processes on the organophosphine fluoride acceptors with substitutions of varying steric hindrance. Using the B3LYP method [36] , [37] , [38] , [39] , [40] , two-step addition-elimination pathways for both F/F isotope exchange and the competing OH/F substitution ( i.e ., hydrolysis) were identified for five representative organophosphine fluorides ( 1 – 5 ). Detailed reaction mechanisms and free energy profiles are shown in Fig. 2 . Such a mechanistic path suggests an inversion of the tetravalent phosphorus after a single F/F exchange. Hence, the overall reactions are not strictly free energy neutral but negligible. The OH/F exchange processes share similar reaction pathways with the exception that [F…H 2 O] − binds with the phosphorus center using its oxygen atom in the first addition step. Fig. 2 Mechanism of H 2 O-resistant 18 F/ 19 F exchange interpreted by free energy parameters. Geometries are optimized at the B3LYP/6-31+G* level of theory, and single point calculations are performed at the CAM-B3LYP/6-311++G** level of theory. Two substituent groups on the phosphorus center are simplified as two large spheres in the molecular structures for clarity. a Reaction pathways and free energy (kcal mol −1 ) profiles for the F/F isotope exchange process of five selected reactant systems. b Reaction pathways and free energy (kcal mol −1 ) profiles for the OH/F exchange process of the same five selected reactant systems Full size image The calculated free energy profiles show that the pentacoordinate intermediates are unstable compared to the initial materials for both F/F isotope exchange and OH/F substitution. A comparison of the relative stabilities of TS1-X and TS2-X (X = 1 – 5 ) to those of TSO1-X and TSO2-X shows that the free energy barriers for the F/F exchange processes were distinctly lower than the corresponding values for the OH/F substitution. The differences in relative free energy values between TS1-X and TSO1-X for the 1 – 5 reaction systems were −3.6, −4.1, −5.1, −7.2, and −4.7 kcal mol −1 , respectively, while those between TS2-X and TSO2-X for the five reaction systems were −5.9, −7.8, −7.1, −8.1, and −4.4 kcal mol −1 , respectively. These results strongly indicate that the F/F isotope exchange is kinetically more favorable than the corresponding OH/F substitution for all of the reactant systems. According to the calculated relative free energies of the transition states, the predicted rates for F/F isotope exchange follow the order of 1 ≈ 2 > 5 > 4 > 3 . In addition, the OH/F substitution processes exhibit endothermic free energy values ( e.g ., ∆G = 2.3–5.1 kcal mol −1 ), suggesting that these processes are neither spontaneous nor thermodynamically favorable. 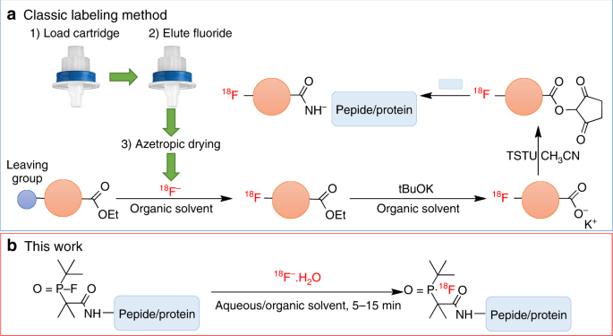Fig. 1 Overview of18F-labeling methods for solvent/heat-sensitive biomolecules.aCommonly used multistep synthetic route beginning with drying of aqueous [18F]F−.bOne-step18F-labeling of biomolecules via an organophosphine fluoride acceptor that allows for efficient labeling with good RCYs (>50%) under mild conditions within 5–15 min Overall, the DFT calculations demonstrate that the 18 F/ 19 F isotope exchange occurs automatically rather than the competing OH/F substitution in terms of both kinetics and thermodynamics (Table 1 ). Table 1 Comparison of flourophosphines with various degrees of steric hindrance Full size table Synthesis of organofluorophosphine fluoride acceptors Next, the designed organofluorophosphine fluoride acceptors were prepared via oxidative coupling between various hydrophosphine oxide and F − . Specifically, dibutylphosphinic fluoride ( 1 ), diphenylphosphinic fluoride ( 2 ), tert -butyl(phenyl)phosphinic fluoride ( 3 ) and benzyl 2-( tert -butylfluorophosphoryl)-2-methylpropanoate ( 4 ) were synthesized from phosphine oxides using the Reformatsky-type reaction [41] , followed by copper-promoted fluorination of phosphine [42] . Compound 1 was found to be difficult to obtain and only 19 F and 31 P NMR spectra were obtained because of its volatility and low yield. Radiochemistry For radiolabeling tests, [ 18 F]F − solution unloaded from a cyclotron target was diluted and added to reaction vials pre-charged with the organofluorophosphine fluoride acceptors. Rapid 18 F-labeling was achieved in high RCYs by 18 F/ 19 F isotope exchange in aqueous or organic solvents without heating. The RCYs were further measured by changing H 2 O ratio from 0 to 95% at graded precursor concentrations and reaction temperatures. For the first try, one-step 18 F-labeling in >95% aqueous solutions was achieved with >50% RCY under mild conditions [31] . As the precursor concentrations and reaction temperatures increased, the RCYs improved significantly. Under the same labeling conditions, [ 18 F] 3 and [ 18 F] 4 were more rapidly labeled with higher yields than [ 18 F] 2 . 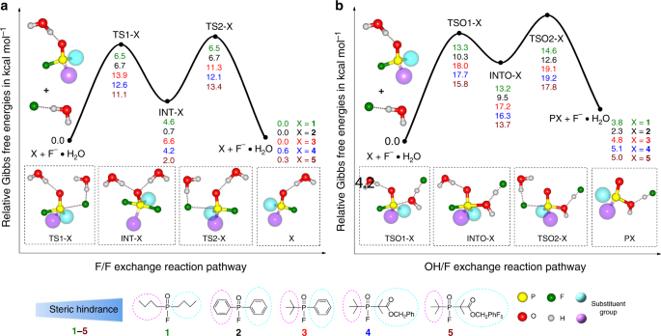Fig. 2 Mechanism of H2O-resistant18F/19F exchange interpreted by free energy parameters. Geometries are optimized at the B3LYP/6-31+G* level of theory, and single point calculations are performed at the CAM-B3LYP/6-311++G** level of theory. Two substituent groups on the phosphorus center are simplified as two large spheres in the molecular structures for clarity.aReaction pathways and free energy (kcal mol−1) profiles for the F/F isotope exchange process of five selected reactant systems.bReaction pathways and free energy (kcal mol−1) profiles for the OH/F exchange process of the same five selected reactant systems 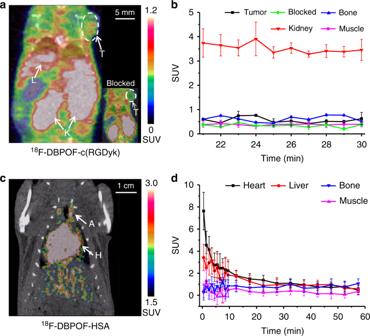Fig. 3 MicroPET/CT imaging with18F-DBPOF-c(RGDyk) and18F-DBPOF-HSA.aA PET image from a dynamic scan with18F-DBPOF-c(RGDyk) in U87MG nude mice bearing gliomablastoma, reconstructed at 23 min post-injection with the tumor (T), live (L), and kidney (K) indicated by white arrows. The inset image in the right corner showed no specific tumor uptake indicated by a white arrow.bTime-activity curves of18F-DBPOF-c(RGDyk) in the tumor, bone, blood, kidney and muscle. Uptake values are presented by means ± standard deviations (n= 3).cA PET image from a 60 min dynamic scan with18F-DBPOF-HAS in healthy female Wistar rats, reconstructed at 60 min post-injection with the heart (H) and artery (A) indicated by white arrows.dTime-activity curves of18F-DBPOF-HSA in the heart, liver, bone and muscle. Uptake values are presented by means ± standard deviations (n= 3). Source data are provided as a Source Data file [ 18 F] 3 and [ 18 F] 4 achieved a 100% labeling yield in dimethyl sulfoxide (DMSO) at 75 °C, as shown in Table 2 . The molar activity of manually labeled [ 18 F] 4 was measured to be 0.01–0.05 Ci μmol −1 (depending on the amount of starting radioactivity, decay-uncorrected) at the end of synthesis. Detailed radiolabeling procedures and calculations are described in the supporting information. Table 2 RCYs of 18 F-labeled fluorophosphine synthons under various conditions Full size table Stability of 18 F-labeled organofluorophosphine In vitro stabilities of [ 18 F] 2 , [ 18 F] 3 , and [ 18 F] 4 in human serum, saline, and ethanol, respectively, are shown in Supplementary Figure 5 . Among these 18 F-labeled fluorophosphines, [ 18 F] 4 exhibited the highest in vivo stability (Table 1 ). During a metabolic stability examination, [ 18 F] 4 remained 100% intact at 2 h post-injection and was more stable than [ 18 F] 3 , which is in good agreement with the predictions from the free energy barrier calculations (Table 1 ). MicroPET/CT imaging with [ 18 F] 4 in healthy ICR mice was then performed to investigate the in vivo metabolic process. No increase in bone uptake was observed up to 120 min post-injection. The radioactivity was primarily concentrated in the bladder and gallbladder over time (see Supplementary Figure 7 ). 2,3,5,6-Tetrafluorophenyl 2-( tert -butylfluorophosphoryl)-2-methylpropanoate (DBPOF-COOC 6 HF 4 , 5 ), a derivative with an activated ester, was synthesized and conjugated to several peptide ligands of clinical interest [43] , [44] to obtain one-step-labeling precursors. Radiosynthesis of 18 F-DBPOF-c(RGDyk) and PET imaging Using a manual labeling procedure, 18 F-DBPOF-c(RGDyk) as a peptide ligand was prepared at an average RCY (the amount of activity in the final product expressed as the percentage of starting activity) of >30% in 25 min with >98% purity after purification with a C-18 solid-phase extraction cartridge. In order to obtain cGMP compliant 18 F-DBPOF-c(RGDyk), we established an automated procedure using a commercial multifunction radiosynthesis module PET-MF-2V-IT-I (Beijing PET Technology, China). The schematic layout of the automated synthesis module is shown in Supplementary Figure 4 . Quality control analysis protocols were established according to the United States Pharmacopeia guidelines for PET radiopharmaceuticals. Average RCY (the amount of activity in the final product expressed as the percentage of starting activity) was 15–25% for the automated procedure. The radiochemical purity of 18 F-DBPOF-c(RGDyk) was confirmed to be >95% by radio-HPLC analysis. The molar activity was measured to be 0.06–0.13 Ci μmol −1 for the product prepared using the automated module, compared to 0.006–0.01 Ci μmol −1 for the manually prepared product. MicroPET/CT imaging data, shown in Fig. 3a , indicated an uptake of 18 F-DBPOF-c(RGDyk) with standardized uptake value (SUV) of 0.76 in U87MG gliomablastoma, and a target to non-target ratio of 2.4. No obvious signal was detected in the tumor as illustrated in the inset image of Fig. 3a , demonstrating that the specific uptake was blocked by DBPOF-c(RGDyk). Fig. 3 MicroPET/CT imaging with 18 F-DBPOF-c(RGDyk) and 18 F-DBPOF-HSA. a A PET image from a dynamic scan with 18 F-DBPOF-c(RGDyk) in U87MG nude mice bearing gliomablastoma, reconstructed at 23 min post-injection with the tumor (T), live (L), and kidney (K) indicated by white arrows. The inset image in the right corner showed no specific tumor uptake indicated by a white arrow. b Time-activity curves of 18 F-DBPOF-c(RGDyk) in the tumor, bone, blood, kidney and muscle. Uptake values are presented by means ± standard deviations ( n = 3). c A PET image from a 60 min dynamic scan with 18 F-DBPOF-HAS in healthy female Wistar rats, reconstructed at 60 min post-injection with the heart (H) and artery (A) indicated by white arrows. d Time-activity curves of 18 F-DBPOF-HSA in the heart, liver, bone and muscle. Uptake values are presented by means ± standard deviations ( n = 3). Source data are provided as a Source Data file Full size image Radiosynthesis of 18 F-DBPOF-HAS and PET imaging Human serum albumin (HSA, 66.5 kDa) is a heat-sensitive globular protein that exhibits high solubility and stability with a plasma half-life of 16–18 h [45] . DBPOF-HSA was prepared by simple conjugation of DBPOF-COOC 6 HF 4 to HAS within 30 min. By manual 18 F-labeling, the RCY (the amount of activity in the final product expressed as the percentage of starting activity) of 18 F-DBPOF-HSA was >5% with molar activity of ~0.03 Ci μmol −1 in shorter synthesis time than other radiofluorination strategies. PET imaging of healthy female Wistar rats was conducted 1 h after intravenous injection of 18 F-DBPOF-HSA. A whole-body PET/CT of a healthy rat 1 h after 18 F-DBPOF-HSA injection through tail vein is demonstrated in Fig. 3c . The heart ventricles the and the peripheral blood vessels are clearly revealed. Other organs can be also observed but with lower activity concentrations than that in the central vessels. Analysis of 18 F-DBPOF-HSA biodistribution in rats showed high retention in blood with SUVs of 2.4 ± 0.6, 1.4 ± 0.7, and 1.0 ± 0.1 at 0.2, 0.5, and 1 h, respectively. The tissue uptake from the microPET/CT experiments agreed well with the biodistribution results at matched time points. These results indicated that the introduction of DBPOF synthon into HSA and subsequent radiolabeling did not affect the structural or functional integrity of HSA. Biomolecules, such as proteins, carbohydrates, and nucleic acids, are excellent vectors for monitoring physiological and biochemical lesions via PET imaging due to their high affinity and high specificity for many pathogenic targets [46] as well as superior biocompatibility. Most of these vectors are soluble and remain intact in water alone or mixed aqueous solvents rather than in organic solvents, while anionic [ 18 F]F − , with its high solvation energy, becomes inactive in the same solvents. Consequently, the direct incorporation of 18 F is challenging, especially in the case of temperature-, pH- and solvent-sensitive macromolecules. Fortunately, efficient aqueous labeling approaches are theoretically feasible by employing highly fluorophilic fluoride acceptors with very low activation energy and high hydrolysis energy for selective fluoro-substitution. Indeed, fluorophosphine fluoride acceptors have been shown to undergo rapid radiofluorination reaction in at least partially aqueous media [10] . Theoretical DFT calculations confirmed that the F/F exchange of organophosphines is more favorable both kinetically and thermodynamically than the OH/F exchange, which is consistent with our experimental findings. The detailed reaction mechanisms and free energy variations were illustrated for the organophosphine labels with five representative reactants. In our calculations, the 1:1 hydrogen-bond complex of H 2 O with F − (F − ·H 2 O) was modeled as a nucleophile to account for the solvation effect of water. Nucleophilic substitution at the tetravalent phosphorus center may occur via either a concerted pathway or a stepwise addition-elimination pathway. The latter method involves a pentavalent adduct intermediate owing to the addition of a nucleophile without the loss of a leaving group. In addition to the spontaneity and aqueous tolerance of these radiolabeling reactions, the compact prothesis configuration and favorable in vivo behavior of the resulting PET tracers are also important. [ 18 F] 2 was found to be unstable at pH 7.4–7.6 in human serum, saline, and ethanol because the steric hindrance of benzene is relatively small. In contrast, [ 18 F] 3 and [ 18 F] 4 exhibited remarkable thermal and hydrolytic stability. The stabilities of 18 F-labeled fluorodiphenylphosphines are consistent with the steric parameters of these compounds, i.e., greater steric hindrance leads to better stability. By virtue of their small size, zero net charge, and negligible decomposition, the physicochemical properties of the 18 F-labeled tracers prepared via the organophosphine fluoride acceptors are similar to those of the unlabeled analogs. Phosphorus compounds are used in many modern homogeneous catalyst systems because the P-X bonds are thermally robust in general and unlikely to break down by transition metals at the catalysis conditions [47] . Fluorophosphines with bulky or electron-withdrawing substituents, such as (C 6 F 5 ) 2 PF, (CF 3 ) 2 PF, and tBu 2 PF, are also found to be thermally stable [48] , [49] , [50] , [51] . Synthesis and screening of more fluorophosphine fluoride acceptors with various leaving groups are continuing in our laboratories. In summary, we have developed a procedure for the radiolabeling of a series of organofluorophosphine biomolecules using 18 F-fluoride. Low activation energy is required for the formation of these P-F bonds in comparison to P-OH bonds. As a result, 18 F-labeling can be performed in aqueous media and high radiochemical yields achieved even at room temperature, and acceptable molar activities that are critical for targeted imaging [52] . This inexpensive, rapid, one-step 18 F-radiolabeling procedure holds great promise for widespread applications in radiopharmaceutical industry to produce a variety of biomolecules as potential PET tracers. Automated radiosynthesis of 18 F-DBPOF-c(RGDyk) No-carrier-added [ 18 F]F − was obtained by bombardment of a H 2 18 O target with 11-MeV protons in a RDS 111 cyclotron (Siemens, Germany) and delivered to the PET-MF-2V-IT-I synthesis module. The aqueous [ 18 F]F − solution (600–1200 mCi) was mixed with a solution of the unlabeled precursor DBPOF-c(RGDyk) (0.8–2.4 mg, 1–3 µmol) in ~0.5 mL of DMSO/H 2 O (1:1, v/v, pH = 7.4) in the reaction vial. The vial was kept at room temperature for 15 min without stirring. The reaction mixture was diluted with 10.0 mL of H 2 O and loaded onto a C18 light cartridge (Waters, USA). The cartridge was flushed twice with 10.0 mL of pure water each to remove the unreacted [ 18 F]F − , then eluted with 1.0 mL ethanol to recover 90–150 mCi of radiochemically pure product collected in a glass vial. This solution was then formulated in 0.9% sodium chloride (9.0 mL) and filtered through a 0.22-µm sterile Millex® GV (vented filter, Millipore, Billerica, MA, USA) into a sterile dose vial (Mallinckrodt, Hazelwood, MO, USA) fitted with a vent needle (Sartorius Stedim Biotech GmbH, Göttingen, Germany). A small sample was removed for quality control analysis. The radiolabeling procedure was repeated at least three times. Detailed HPLC profiles and procedure for molar activity measurements are presented in the Supplementary Information. Radiosynthesis of 18 F-DBPOF-HAS DBPOF-HAS (2–3 mg) was dissolved in 150 μL of 0.01 M phosphate buffered saline (pH = 7.36) in a glass vial. Aqueous [ 18 F]F − solution (50 μL, 30–50 mCi) unloaded from the cyclotron target was added to the reaction vial. The vial was gently shaken at room temperature for 15 min. With the reaction impurities ( i.e ., free [ 18 F]F − ) removed by a radio-HPLC equipped with a Xtimate SEC-300 column (Welch, China), 1.5–2.8 mCi of the desired product was collected. A small sample was removed for quality control analysis. Radiochemical purity was measured by a radio-HPLC with a Xtimate SEC-300 column. The radiolabeling was repeated at least three times. Detailed analytical HPLC procedures are presented in the Supplementary Information. MicroPET/CT imaging All animal studies were performed under the animal use and care regulations approved by Center of Animal Care and Use Committee, Xiamen University. Dynamic microPET-CT scans were acquired by an Inveon microPET/CT (Siemens, Germany). Reconstruction of PET images was performed with 3D OPMAP algorithm. Reporting summary Further information on experimental design is available in the Nature Research Reporting Summary linked to this article.